Cell division and targeted cell cycle arrest opens and stabilizes basement membrane gaps Large gaps in basement membrane (BM) occur during organ remodelling and cancer cell invasion. Whether dividing cells, which temporarily reduce their attachment to BM, influence these breaches is unknown. Here we analyse uterine–vulval attachment during development across 21 species of rhabditid nematodes and find that the BM gap that forms between these organs is always bounded by a non-dividing vulval cell. Through cell cycle manipulation and live cell imaging in Caenorhabditis elegans , we show that actively dividing vulval cells facilitate enlargement of this breach by promoting BM movement. In contrast, targeted cell cycle arrest halts BM movement and limits gap opening. Further, we demonstrate that the BM component laminin accumulates at the BM gap edge and promotes increased integrin levels in non-dividing vulval cells, stabilizing gap position. Together, these studies reveal that cell division can be used as a mechanism to regulate BM breaches, thus controlling the exchange of cells between tissues. The basement membrane (BM) is an ancient specialized extracellular matrix that arose at the emergence of multicellular animals [1] . Composed of a thin, dense, sheet-like structure engineered on polymeric laminin and type IV collagen networks, BM surrounds most tissues, providing structural integrity and forming one of the main barriers to motile cells [2] . The evolution of BM was likely vital in supporting tissue-level complexity and the three-dimensional (3D) multicellular metazoan body plan [3] , [4] . Although critical for multicellular complexity, during cell migration and organ remodelling large de novo gaps in BM are generated to enable the escape of cells from tissues. For example, during chick gastrulation a large gap in the BM is created that facilitates the migration of mesodermal cells [5] , [6] . Before gastrulation during early mouse development, a large BM-breaching event is required to form the distal visceral endoderm [7] . BM openings also occur during Drosophila metamorphosis when internal imaginal discs break through epidermal BM [8] . Formation of large breaks in epithelial BMs is also a defining feature in the transition from benign to metastatic potential in tumours and enables tumour cell spread into the interstitial matrix and vasculature [9] , [10] , [11] . In all of these contexts, BM breaches occur in growing tissues with proliferating cells. Although the BM is often thought of as a static matrix, recent optical labelling studies have shown that the BM can move and shift its position [12] , [13] . Thus, it remains an important question to understand whether actively dividing cells, which briefly reduce or lose their attachment to BM [14] , [15] , might be a mechanism to regulate BM gap openings. Despite profound basic and clinical significance, the mechanisms regulating BM breaches has remained poorly defined, largely due to the lack of in vivo models to study cell-BM interactions [16] . Caenorhabditis elegans uterine–vulval attachment is a visually and experimentally tractable model to functionally dissect the mechanisms involved in the creation and stabilization of BM gaps [13] , [17] . A specialized uterine cell, the anchor cell (AC), initiates uterine–vulval connection by breaching BM and invading between the centrally located vulval precursor cells (VPCs) [17] , [18] . Following AC invasion, the VPCs continue their divisions, expand in size and invaginate. Optical highlighting of BM components and laser-directed killing of cells has shown that VPC invagination generates forces that physically moves the BM, opening the BM gap wider independent of large-scale proteolysis and degradation [13] , [19] . The BM slides over the invaginating central VPCs (F and E cells) and in an integrin-dependent fashion halts its displacement on the vulval D cells ( Fig. 1a ) [13] . The mechanisms that facilitate the precise movement and stabilization of BM over the D cells are not known. 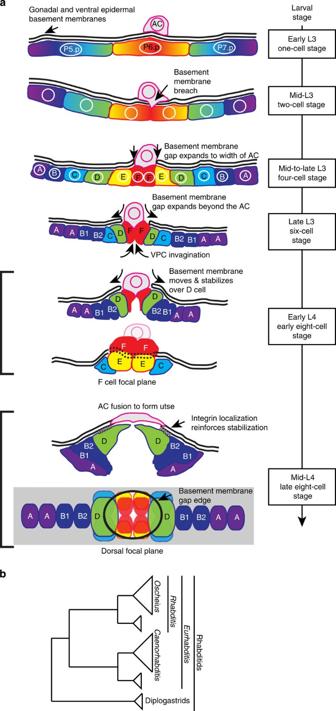Figure 1:C. elegansuterine–vulval attachment and rhabditid nematode phylogeny. (a) Stages of uterine–vulval attachment inC. elegans. At the P6.p one-cell stage (early L3 larval stage) the VPCs (P5.p–P7.p) are separated from the uterine AC (magenta, other uterine cells are not shown for simplicity) by the gonadal and ventral epidermal BMs (black). At the P6.p two-cell stage (mid-L3), the AC initiates BM breach. At the P6.p six-cell stage (late L3), the E and F cells invaginate, the E cells divide (the daughter cells move laterally and are out of the plane of focus) and the BM gap expands. At the early P6.p eight-cell stage (early L4), the VPCs invaginate further and the interior F cells have completed their terminal division (the daughters also divide laterally). By this time the BM gap boundary expands over the E and F cells (shown in a lateral focal plane (the F cell focal plane)) and stabilizes over the D cells. At the late P6.p eight-cell stage (mid-L4) the AC fuses with the neighbouring ventral uterine cells to form the utse and integrin is upregulated at the D cell–BM gap position. A dorsal view indicates the position of the VPCs at this time. (b) Summary phylogeny of the rhabditid nematodes in this study (seeSupplementary Fig. 3afor complete phylogeny based on refs20,21,22,23). Figure 1: C. elegans uterine–vulval attachment and rhabditid nematode phylogeny. ( a ) Stages of uterine–vulval attachment in C. elegans . At the P6.p one-cell stage (early L3 larval stage) the VPCs (P5.p–P7.p) are separated from the uterine AC (magenta, other uterine cells are not shown for simplicity) by the gonadal and ventral epidermal BMs (black). At the P6.p two-cell stage (mid-L3), the AC initiates BM breach. At the P6.p six-cell stage (late L3), the E and F cells invaginate, the E cells divide (the daughter cells move laterally and are out of the plane of focus) and the BM gap expands. At the early P6.p eight-cell stage (early L4), the VPCs invaginate further and the interior F cells have completed their terminal division (the daughters also divide laterally). By this time the BM gap boundary expands over the E and F cells (shown in a lateral focal plane (the F cell focal plane)) and stabilizes over the D cells. At the late P6.p eight-cell stage (mid-L4) the AC fuses with the neighbouring ventral uterine cells to form the utse and integrin is upregulated at the D cell–BM gap position. A dorsal view indicates the position of the VPCs at this time. ( b ) Summary phylogeny of the rhabditid nematodes in this study (see Supplementary Fig. 3a for complete phylogeny based on refs 20 , 21 , 22 , 23 ). Full size image As C. elegans is just one of many free-living nematode species, there exists a rich comparative framework with a well-resolved phylogeny [20] , [21] , [22] , [23] to identify evolutionary mechanisms that mediate BM remodelling during uterine–vulval attachment. Vulval development has been examined in over 50 species of rhabditid nematodes and is an excellent model of comparative organogenesis [20] , [24] , [25] , [26] , [27] , [28] . These studies have demonstrated examples of characters that show a surprising amount of evolutionary change, likely due to a high level of developmental system drift or a large range of variation in the development of homologous conserved structures [20] , [28] . At the same time, several characters are invariant, suggesting that they may be under a ‘developmental constraint’ and directed by biased deterministic or purifying selective pressure for a specific patterning or morphogenetic function [20] , [29] . To investigate potential evolutionarily conserved mechanisms that underlie BM gap formation we have examined uterine–vulval attachment in C. elegans and 19 additional species of Eurhabditid nematodes and a diplogastrid outgroup, Pristioncus pacificus , which last shared a common ancestor estimated at 280–430 million years ago [30] . We find that the AC initiates uterine–vulval connection in all species examined by breaching the BM and that invasion always occurs before vulval cell invagination. Similar to C. elegans , BM gap expansion followed vulval invagination in all species and halted over the D cell. Notably, the D cell is the only vulval cell that precociously exits the cell cycle in all rhabditid species surveyed [20] . This ‘developmental constraint’ suggested that the D cells might be under selective pressure to limit BM gap expansion. Utilizing cell cycle manipulation in C. elegans we show that extra division cycles within the D lineage result in additional BM movement and expansion of the BM gap beyond the D cell descendants. Conversely, inhibition of the interior E and F vulval cell divisions limited BM movement and resulted in a narrower opening. Analysis of the VPC–BM interaction revealed that the dividing vulval cells reduce or lose contact with the BM, providing a mechanism that allows movement of the BM to the neighbouring cell. Further, we find that increased laminin levels at the lip of the BM gap promote higher levels of INA-1/PAT-3 (integrin) in post-mitotic cells, stabilizing the BM gap position. This evolutionary-cell biological study identifies cell division and targeted cell cycle exit as a new mechanism to expand and stabilize BM gaps that can be used to build organs and facilitate the exchange of cells between tissues. Summary of uterine–vulval attachment and BM gap opening Before uterine–vulval attachment the uterine AC is positioned over the P6.p VPC, which sits between the P5.p and P7.p VPCs during the early L3 stage of larval development ( Fig. 1a ). The AC initiates uterine–vulval connection by breaching the juxtaposed gonadal and ventral epidermal BMs and contacting the daughters of P6.p (P6.p two-cell stage) [17] . We have shown previously that following AC invasion, the two BMs become fused at the borders of the invading AC where they form a continuous BM throughout uterine–vulval attachment ( Fig. 1a ) [13] . AC invasion is highly stereotyped and is tightly coordinated with P6.p divisions and stages of larval development. AC breach is first detectable under high magnification (× 1,000) using differential interference contrast (DIC) microscopy as a small break in the phase dense line underneath the AC [19] . This phase dense line correlates with immunolocalization and functional translational GFP fusions to the main structural components of the BM, laminin and type IV collagen [13] , [17] , [31] . Shortly after the second division of P6.p (P6.p four-cell stage, Fig. 1a ), the BM gap expands to the width of the AC. Following AC invasion at the late L3 stage, the VPCs (arrayed linearly from anterior to posterior as ABCDEFFEDCBA) invaginate. Vulval invagination is accompanied by cell division in all VPCs except the D cells. Invagination and expansion of the vulval cells exert force on the overlying BM, which opens the gap wider by shifting the BM beyond the boundary of the AC and onto the vulD precursor cells by the P6.p eight-cell stage (early L4, Fig. 1a ) [13] . In the mid-L4 stage, integrin is upregulated at the D cell–BM boundary, stabilizing BM gap position [13] . At this time the AC fuses with neighbouring ventral uterine cells and forms the syncytial utse cell ( Fig. 1a ) [18] . BM gap opening enables direct contact between the uterine uv1 cells and the utse with the underlying vulF and vulE cells to form the mature uterine–vulval connection [32] , [33] , [34] . BM breach occurs before vulval cell invagination To compare mechanisms of BM remodelling during uterine–vulval attachment in nematodes, we investigated AC behaviour in 20 Eurhabditid nematodes (including C. elegans ) and the diplogastrid outgroup, Pristionchus pacificus ( Fig. 1b ). Using DIC microscopy we scored for BM breach in relation to the divisions of the P6.p cell (corresponding to the P6.p one-cell, two-cell, four-cell stage; n ⩾ 50 animals examined for each stage, Fig. 2a,b ; Supplementary Fig. 1 and Supplementary Table 1 ). Notably, in all species we found that the AC initiated uterine–vulval attachment through a BM invasion event. The timing of the BM breach varied between the late P6.p one-cell stage to the early P6.p four-cell stage. Eight species showed an initial BM breach between the late P6.p one-cell stage and early P6.p two-cell stage (8/21 species examined) and the remainder breached between the late P6.p two-cell stage and early P6.p four-cell stage (13/21 species examined; Fig. 2b ). One common feature of invasion was that in all species examined the AC invaded before initiation of vulval invagination at the late P6.p four-cell stage ( Fig. 2b ). 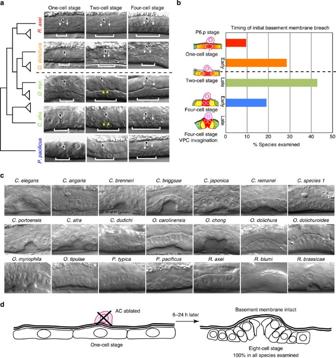Figure 2: The rhabditid nematode AC breaches the BM and initiates uterine–vulval attachment before vulval invagination. (a) DIC microscopy of five representative species of rhabditid nematodes. DIC micrographs depict the position of the AC (black arrowhead), width of the BM breach (yellow arrowheads, partial invasion; white arrows, full invasion) and division stage of P6.p (white brackets) at the P6.p one- (left), two- (middle) and four-cell stage (right;n⩾50 animals examined for each stage and species; seeSupplementary Table 1for scoring data andSupplementary Fig. 1for DIC micrographs of all 21 rhabditid species). Colours differentiate between those species that invade ‘early’ (in relation to P6.p divisions) at the late P6.p one- (red text) or the early two-cell stage (orange) and those that invade ‘late’ at the late P6.p two- (green) and the early P6.p four-cell stage (blue). Phylogeny depicts evolutionary relationships between study species (seeSupplementary Fig. 3afor complete phylogeny, based on refs20,21,22,23). (b) Bar graph depicting the percent of species that show an initial BM breach relative to the divisions of the P6.p cell. Dashed line at the P6.p two-cell stage delineates division between the two main groups in the timing of AC invasion, with coloured bars matching the corresponding species shown in (a). (c) For all rhabditid nematodes surveyed (n=10 animals for each), laser ablation of the AC at the P6.p one-cell stage, before a detectable BM breach, resulted in an intact BM (schematized ind). Scale bars, 5 μm. Figure 2: The rhabditid nematode AC breaches the BM and initiates uterine–vulval attachment before vulval invagination. ( a ) DIC microscopy of five representative species of rhabditid nematodes. DIC micrographs depict the position of the AC (black arrowhead), width of the BM breach (yellow arrowheads, partial invasion; white arrows, full invasion) and division stage of P6.p (white brackets) at the P6.p one- (left), two- (middle) and four-cell stage (right; n ⩾ 50 animals examined for each stage and species; see Supplementary Table 1 for scoring data and Supplementary Fig. 1 for DIC micrographs of all 21 rhabditid species). Colours differentiate between those species that invade ‘early’ (in relation to P6.p divisions) at the late P6.p one- (red text) or the early two-cell stage (orange) and those that invade ‘late’ at the late P6.p two- (green) and the early P6.p four-cell stage (blue). Phylogeny depicts evolutionary relationships between study species (see Supplementary Fig. 3a for complete phylogeny, based on refs 20 , 21 , 22 , 23 ). ( b ) Bar graph depicting the percent of species that show an initial BM breach relative to the divisions of the P6.p cell. Dashed line at the P6.p two-cell stage delineates division between the two main groups in the timing of AC invasion, with coloured bars matching the corresponding species shown in ( a ). ( c ) For all rhabditid nematodes surveyed ( n =10 animals for each), laser ablation of the AC at the P6.p one-cell stage, before a detectable BM breach, resulted in an intact BM (schematized in d ). Scale bars, 5 μm. Full size image Available antibodies to BM components fail to crossreact with high specificity in other non-model rhabditid nematodes. Thus, to confirm that our DIC imaging of AC invasion reflected BM removal we injected rhodamine-labelled dextran into the body cavity of three species ( C. elegans , O. carolinensis and P. pacificus ). From examination of colocalization of dextran in a C. elegans strain containing laminin::GFP, we have found that dextran localizes to BM, thus clearly outlining breaches and BM boundaries ( Supplementary Fig. 2a ). In all three species examined, rhodamine dextran staining confirmed the timing of AC invasion by DIC optics ( Fig. 2a,b ; Supplementary Fig. 2a–c ). Taken together, our observations indicate that AC invasion through BM initiates uterine–vulval attachment across rhabditid nematode evolution and suggest a necessity for invasion before vulval invagination. The AC is required to initiate BM breach in rhabditids The AC is the only cell capable of breaching the BM during C. elegans uterine–vulval attachment [13] . To determine whether the AC is required to initiate the BM breach in species other than C. elegans , we laser-ablated the AC at the P6.p one-cell stage several hours before invasion in the 21 rhabditid nematodes investigated. Examination of the BM by DIC microscopy during the mid-L4 stage ( Fig. 2c,d ) revealed an intact BM and a failure to connect the uterine and vulval tissues in all species ( Fig. 2c,d ; n =10 for each species). Thus, our laser ablation data suggest that the AC appears to be the only cell able to breach the BM to initiate the uterine–vulval connection. The BM gap stabilizes over the D cells in rhabditids We have previously shown that following AC invasion in C. elegans , the gap in the BM widens. This expansion occurs through BM movement over the invaginating vulval cells in the late L3 stage followed by stabilization of the gap boundary over the vulD precursor cells by the early L4 stage ( Fig. 1a ) [13] . To determine whether BM gap position is flexible or fixed across evolutionary time, we examined the location of the gap in the 20 other rhabditid nematode species. Strikingly, despite species-specific variation in the width of the BM gap (likely due to differences in cell size between species [35] ) at the late P6.p eight-cell stage ( Supplementary Fig. 3b ), in all 20 species the BM gap boundary similarly resided over the vulD precursors ( Fig. 3a ; Supplementary Fig. 2a–c ). While there have been many changes in cell division patterns across rhabditid nematode vulval evolution, the D cells are unique, as they are the only vulval cells that do not divide in all species examined during vulval invagination [20] . The strong correlation with BM gap stabilization and cell cycle exit suggested that the cell cycle in D cells might be uniquely regulated to halt BM hole expansion. 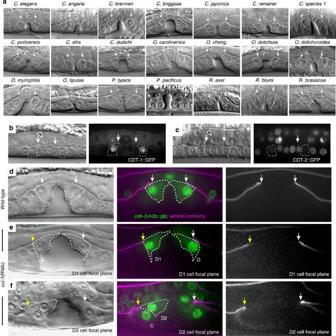Figure 3: VulD precursor cell cycle exit stabilizes BM gap position. (a) DIC micrographs ofC. elegansand the 20 rhabditid nematode species at the P6.p eight-cell stage show that the BM gap has stabilized over the undivided D cells (dashed lines) in all species (n=15 for each species). DIC micrographs depict the position of the AC (black arrowheads) and width of the BM breach (white arrows, seeSupplementary Fig. 2for dextran labelling of the BM in representative species andSupplementary Fig. 3bfor BM gap measurements). (b,c) DIC images (left) and corresponding confocal sections (right) of cell cycle reporters (b) CDT-1::GFP (nuclear localized in G1/G0) and (c) CDT-2::GFP (nuclear localized in mitotic cells) at the P6.p four-cell stage, shortly after the terminal division of the D cell (dashed lines). (d–f) DIC images (left), confocal sections of BM labelled with laminin::mCherry (magenta, middle) and the nuclei of C and D cells labelled withcdh-3>H2B::GFP(green, middle), and BM fluorescence alone (right) in mid-L4 animals. (e,f) RNAi depletion of the G1/S phase regulatorcul-1resulted in an additional D cell division (transverse division, labelled D1 (e) and D2 (f) in a lateral focal plane (D2 cell focal plane)). The BM boundary expanded beyond the two D daughter cells and resided over the B2 and C cells (yellow arrow,eandf,n=7/8 cases). Scale bars, 5 μm. Figure 3: VulD precursor cell cycle exit stabilizes BM gap position. ( a ) DIC micrographs of C. elegans and the 20 rhabditid nematode species at the P6.p eight-cell stage show that the BM gap has stabilized over the undivided D cells (dashed lines) in all species ( n =15 for each species). DIC micrographs depict the position of the AC (black arrowheads) and width of the BM breach (white arrows, see Supplementary Fig. 2 for dextran labelling of the BM in representative species and Supplementary Fig. 3b for BM gap measurements). ( b , c ) DIC images (left) and corresponding confocal sections (right) of cell cycle reporters ( b ) CDT-1::GFP (nuclear localized in G1/G0) and ( c ) CDT-2::GFP (nuclear localized in mitotic cells) at the P6.p four-cell stage, shortly after the terminal division of the D cell (dashed lines). ( d – f ) DIC images (left), confocal sections of BM labelled with laminin::mCherry (magenta, middle) and the nuclei of C and D cells labelled with cdh-3>H2B::GFP (green, middle), and BM fluorescence alone (right) in mid-L4 animals. ( e , f ) RNAi depletion of the G1/S phase regulator cul-1 resulted in an additional D cell division (transverse division, labelled D1 ( e ) and D2 ( f ) in a lateral focal plane (D2 cell focal plane)). The BM boundary expanded beyond the two D daughter cells and resided over the B2 and C cells (yellow arrow, e and f , n =7/8 cases). Scale bars, 5 μm. Full size image The D cell exits the cell cycle shortly after its birth To further explore the role of the D cells in BM gap positioning we turned to C. elegans , where experimental manipulations using transgenics, RNAi and genetics are all available. We first examined the regulation of the timing of cell cycle exit in the D cells by generating transgenic C. elegans animals bearing integrated arrays of the genomic locus of the DNA licensing factor cdt -1 fused to GFP. CDT-1 is required for the recruitment of the MCM2-7 helicase to replication origins during the G1 phase of the cell cycle, and its nuclear localization is a marker for cells in the G1/G0 phase [36] , [37] . In contrast, CDT-2, a member of the E3 ubiquitin ligase complex that removes CDT-1 during S phase is nuclear in actively dividing cells [38] . Examination of CDT-1::GFP revealed specific nuclear localization in both D cells as soon as they were born at the P6.p four-cell stage ( Fig. 3b ; n =15/15 animals). Further, this correlated with loss of the nuclear CDT-2::GFP in these same cells, which was expressed and localized to the nucleus of the remaining mitotic VPCs ( Fig. 3c ; n =15/15 animals). We conclude that the D cell in C. elegans undergoes a precisely regulated early cell cycle exit into a G1/G0 state. Inappropriate division of D cells cause BM gap overexpansion Our observations indicated that cell cycle exit of the vulD precursors might regulate BM gap position. To test this idea we drove the D cell into an extra round of division by depleting cul-1 , the C. elegans cullin ortholog. Cul-1 is a negative regulator of the G1/S phase transition, and loss of cul-1 activity results in excess VPC divisions [39] , [40] . We examined cell divisions in cul-1 RNAi-depleted animals using a nuclear VPC marker, cdh -3>H2B::GFP and followed BM position with a functional laminin tagged with mCherry (laminin::mCherry; Fig. 3d–f ). We took advantage of the mosaic penetrance of RNAi in the VPCs to identify animals where only one D cell had inappropriately divided. Notably, in cases with an isolated mitotic D cell, we found an overexpansion of the BM gap boundary past the D daughter cells in most animals ( n =7/8 animals; Fig. 3e,f ), while extra divisions of C, F or E cells failed to alter the BM gap boundary over the D cell ( n =4/4 C, 3/3 E, 1/1 F). These results indicate that early cell cycle exit of the D cell stabilizes the position of the BM gap boundary. The BM moves during E and F cell divisions During invasion, the AC physically displaces the BM, leaving the BM gap border initially either over the E or F cells at the P6.p four-cell stage ( Fig. 1a ) [19] . In C. elegans , the central E and F vulval cells divide during BM sliding. To determine whether these divisions might facilitate BM movement, we compared the timing of E and F vulval cell divisions (using both a cytoplasmic ( egl-17 >GFP) and membrane-bound ( unc-62> GFP::CAAX) GFP expressed in the vulval cells) to the precise movement of the BM gap boundary (laminin::mCherry; Fig. 4 ; Supplementary Fig. 4 ). Owing to the variable nature of the BM gap position over the E or F cells after AC invasion, we scored the initial boundary over E and F cells together (‘E/F’, 26/26 cases; Fig. 4a , Supplementary Fig. 4 and Supplementary Table 2a ). During the late P6.p four-cell stage the E and F cells initiated vulval invagination, changed shape and reduced contact with the BM ( Fig. 4b ). Occasionally, the BM moved and the gap expanded to the D cell at this time (11/56 cases; Fig. 4b ). During invagination, the E cells divide first, resulting in a brief P6.p six-cell stage. During division, the E cells rounded and reduced (and possibly lost) contact with the overlying BM ( Fig. 4c , inset). After the E division was completed (and the daughter cells moved to the left and right sides of the D cell) the BM gap edge resided 56% of the time over the D cells (28/50 cases) and 44% on the now neighbouring F cells (22/50 cases; Fig. 4d ). The F cells similarly rounded during mitosis and appeared to have greatly reduced (and possibly no) contact with overlying BM ( Fig. 4e , inset). After completion of the F cell division, the BM gap boundary resided over the D cells in all cases (32/32 cases; Fig. 4f ) and remained stabilized here through the late P6.p eight-cell stage (40/40 cases; Fig. 4g ). Thus, the edge of the expanding BM gap primarily moves onto the D cell during E and F cell divisions, when these dividing vulval cells reduce contact with the BM. Taken together, these observations suggest that E and F divisions facilitate BM movement to the neighbouring non-dividing D cell. 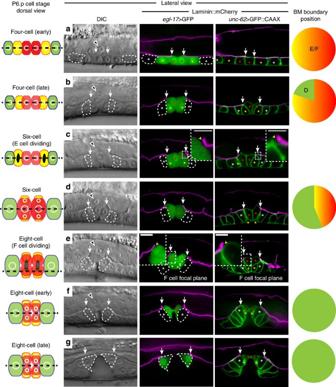Figure 4: E and F vulval divisions correlate with BM gap expansion. (a–g) DIC micrographs (left) and confocal microscopy images of BM (laminin::mCherry, magenta, middle and right) and vulval cells (egl-17>GFP, expressed initially in E and F and then D, cytoplasmic green, middle;unc-62>GFP::CAAX, expressed in all vulval cells, membrane green, right) at the P6.p four- through eight-cell stages. Dorsal schematics (far left) indicate the position of the VPCs at each developmental stage with the dashed black line denoting the location of the single lateral confocal slice depicted by the corresponding micrographs (right, seeSupplementary Fig. 4for corresponding confocal projections of the ventral view at each stage). Black arrowheads indicate the AC and white arrows indicate the BM gap boundary (seeSupplementary Fig. 4for BM gap measurements). Dashed lines (left and middle) and white asterisks (middle and right) indicate D cell position, yellow asterisks indicate E cell position and red asterisks indicate F cells. (a–g) Pie charts depict BM gap position at the P6.p four- through eight-cell stages,n=26, 56, 50, 32 and 40 cases observed, respectively, for each stage (seeSupplementary Table 2afor scoring data). (c,e) Insets depict reduction of BM contact (yellow arrowheads) during E (c) and F (e) cell division. Scale bars, 5 μm. Figure 4: E and F vulval divisions correlate with BM gap expansion. ( a – g ) DIC micrographs (left) and confocal microscopy images of BM (laminin::mCherry, magenta, middle and right) and vulval cells ( egl-17>GFP , expressed initially in E and F and then D, cytoplasmic green, middle; unc-62>GFP::CAAX , expressed in all vulval cells, membrane green, right) at the P6.p four- through eight-cell stages. Dorsal schematics (far left) indicate the position of the VPCs at each developmental stage with the dashed black line denoting the location of the single lateral confocal slice depicted by the corresponding micrographs (right, see Supplementary Fig. 4 for corresponding confocal projections of the ventral view at each stage). Black arrowheads indicate the AC and white arrows indicate the BM gap boundary (see Supplementary Fig. 4 for BM gap measurements). Dashed lines (left and middle) and white asterisks (middle and right) indicate D cell position, yellow asterisks indicate E cell position and red asterisks indicate F cells. ( a – g ) Pie charts depict BM gap position at the P6.p four- through eight-cell stages, n =26, 56, 50, 32 and 40 cases observed, respectively, for each stage (see Supplementary Table 2a for scoring data). ( c , e ) Insets depict reduction of BM contact (yellow arrowheads) during E ( c ) and F ( e ) cell division. Scale bars, 5 μm. Full size image Blocking E and F cell divisions halts BM gap expansion If E and F cell divisions promote BM movement onto the D cells, we hypothesized that blocking their terminal division would prematurely halt BM gap expansion. To test this hypothesis, we expressed a functional GFP fusion to CKI-1 (p27 KIP1 ortholog), a negative regulator of the G1/S phase transition, in the E and F cells at the P6.p four-cell stage ( cdh-3> CKI-1::GFP; Fig. 5a ) [41] . At the late P6.p four-cell stage, the CKI-1::GFP-expressing E cells failed to initiate division (22/22 cases) and the BM boundary remained over the E or F cells (22/22 cases; Fig. 5b ; Supplementary Table 2b ). By the late L3 stage (equivalent to the P6.p ‘six-cell’ stage) the BM gap resided over the E or F cells in most cases (54/56 cases; Fig. 5c ). F cell divisions were also blocked by cdh-3> CKI-1::GFP (93/93 cases), and both at the early and mid-L4 stages (equivalent to the P6.p ‘eight-cell’ stage) the BM primarily stabilized over the non-dividing E/F cells (46/52 and 32/41 cases respectively; Fig. 5d,e ) rather than over the D cell (compare to Fig. 4g ). We conclude that vulval cell divisions promote BM movement, thus allowing gap expansion, while cell cycle exit limits BM sliding and halts further breach opening. 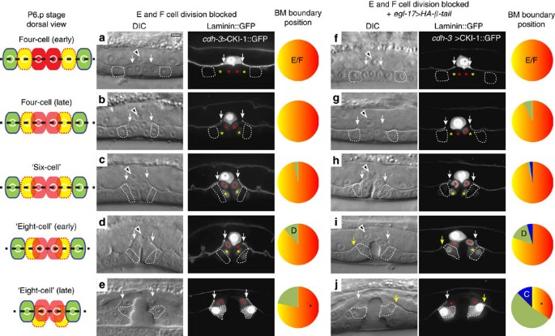Figure 5: Blocking E and F divisions halts BM gap movement in an integrin-dependent fashion. (a–j) DIC micrographs (left) and corresponding confocal sections of the BM (laminin::GFP, right). Dorsal schematics (far left) indicate the position of the VPCs at each developmental stage with the dashed black line denoting the location of the single lateral confocal slice depicted by the corresponding micrographs (right). Black arrowheads indicate position of the AC, white arrows delineate the BM gap, dashed lines, yellow and red asterisks indicate the D, E and F cells, respectively. (a–j) Pie charts depict BM gap position at the P6.p four- through eight-cell stages,n=40, 22, 56, 52, 41, 28, 14, 42, 46 and 32 cases observed for each stage, respectively (seeSupplementary Fig. 5for BM gap measurements andSupplementary Tables 2b,cfor scoring data). (a–e) Expression ofcdh-3>CKI-1::GFP (right) blocked the terminal division of the E and F cells (c,d) and inhibited BM gap expansion beyond these cells. (f–j) Expression of a dominant negative PAT-3 β-integrin construct (HA-β-tail) in the C-F cells (egl-17>HA-β-tail, expressed most strongly in the vulE and vulF precursors) resulted in a progressive overexpansion of the BM gap boundary when E and F cell division was blocked by expression ofcdh-3>CKI-1::GFP (yellow arrows). (j) By the mid-L4 stage, the BM gap boundary expanded beyond the E and F cells 66% of the time (*P<0.0002;n=32, Fisher’s exact test as compared with (e,n=41)). Scale bar, 5 μm. Figure 5: Blocking E and F divisions halts BM gap movement in an integrin-dependent fashion. ( a – j ) DIC micrographs (left) and corresponding confocal sections of the BM (laminin::GFP, right). Dorsal schematics (far left) indicate the position of the VPCs at each developmental stage with the dashed black line denoting the location of the single lateral confocal slice depicted by the corresponding micrographs (right). Black arrowheads indicate position of the AC, white arrows delineate the BM gap, dashed lines, yellow and red asterisks indicate the D, E and F cells, respectively. ( a – j ) Pie charts depict BM gap position at the P6.p four- through eight-cell stages, n =40, 22, 56, 52, 41, 28, 14, 42, 46 and 32 cases observed for each stage, respectively (see Supplementary Fig. 5 for BM gap measurements and Supplementary Tables 2b,c for scoring data). ( a – e ) Expression of cdh-3 >CKI-1::GFP (right) blocked the terminal division of the E and F cells ( c , d ) and inhibited BM gap expansion beyond these cells. ( f – j ) Expression of a dominant negative PAT-3 β-integrin construct (HA-β-tail) in the C-F cells ( egl-17>HA-β-tail , expressed most strongly in the vulE and vulF precursors) resulted in a progressive overexpansion of the BM gap boundary when E and F cell division was blocked by expression of cdh-3 >CKI-1::GFP (yellow arrows). ( j ) By the mid-L4 stage, the BM gap boundary expanded beyond the E and F cells 66% of the time (* P <0.0002; n =32, Fisher’s exact test as compared with ( e , n =41)). Scale bar, 5 μm. Full size image Evolutionary loss of E cell division affects BM gap position Our initial phylogenetic survey of BM gap opening showed that for all 21 species of rhabditid nematodes examined, the BM gap was bounded on the non-mitotic D cell ( Fig. 3a ). Given that forced cell cycle exit in E and F cells stopped BM gap expansion in C. elegans , we wanted to determine whether the natural loss of either of these cell divisions in a nematode lineage would limit BM gap expansion. The diplogastrid P. pacificus has lost the terminal F cell division. Examination of BM positioning, however, revealed that at the P6.p four-cell stage the BM was already lost over the F cells ( Supplementary Fig. 2c ; 36/36 cases observed). This suggests that in P. pacificus F cell divisions are not required to shift the BM, as the AC removes the BM over the F cells during invasion (unlike C. elegans ; Fig. 4 ). Thus, we examined a species more distantly related to our study group, Bursilla sp. (PS1179), one of several Mesorhabditid species in which the E cells do not divide (see Supplementary Fig. 3a for phylogenetic relationships) [20] . We utilized rhodamine dextran body cavity injections to visualize the BM gap boundary and found that at the P6.p six-cell stage (note, there is no eight-cell stage), the BM gap resided over the vulE precursors ( n =5/5 animals; Supplementary Fig. 2d ). Thus, early cell cycle exit of the E cells within a nematode lineage may limit BM gap opening. Integrin mediates BM gap stabilization after cell cycle exit We next wanted to determine how non-dividing cells adhere to the BM. The BM gap is stabilized over the vulD precursors at the P6.p eight-cell stage by the integrin heterodimer INA-1/PAT-3 (ref. 13 ). To determine whether the non-dividing E and F cells (expressing cdh-3> CKI-1::GFP) also stabilize the gap using INA-1/PAT-3, we perturbed integrin function specifically within the vulval cells using a dominant negative integrin β-subunit PAT-3 construct expressed most strongly in the vulE and F precursors ( egl-17 >HA-β-tail [13] ; Figs. 4 and 5f–j ). Loss of integrin signalling in these vulval cells resulted in dramatic BM gap boundary expansion past the non-dividing E and F cells by the mid-L4 stage (21/32 cases, Fig. 5j ; P <0.0002, Fisher’s exact test; Supplementary Fig. 5 and Supplementary Table 2c ). We conclude that non-dividing vulval cells require integrin to limit BM gap opening. Laminin recruits integrin and stabilizes BM gap position An increased level of INA-1/PAT-3 integrin over the vulD precursor cells stabilizes BM gap position [13] . We were next interested in understanding the mechanism underlying this increase. We found that PAT-3::GFP (which when expressed without INA-1 is unable to be secreted to the cell surface [42] ) localized uniformly to the VPCs throughout vulval development ( Supplementary Fig. 6 ), indicating that differential expression is not likely driving increased integrin levels at the D cell–BM interface. We noted during our observations that increased levels of laminin also resided at the BM gap edge ( Fig. 6a ). We quantified laminin::mCherry enrichment over developmental time and discovered that the increased concentration of laminin at the gap edge originated from the AC invasion event, where the AC displaces BM during invasion ( Supplementary Fig. 7 ) [19] . The BM component laminin has been shown to interact with specific integrins in a variety of contexts to promote adhesion to the extracellular matrix [43] , [44] . Thus, we hypothesized that increased laminin at the gap edge might act as a signal for enrichment of INA-1/PAT-3, an integrin predicted to be most similar to vertebrate laminin-binding integrins [45] . To examine this possibility, we first quantified the fluorescence intensity of functional laminin (laminin::mCherry) and integrin (INA-1,PAT-3::GFP [42] ) reporters before and during gap stabilization ( Fig. 6a–c ; Supplementary Fig. 7 ). Laminin::mCherry localization was enriched at the edge of the BM gap from the time of AC invasion throughout vulval development, such that by the P6.p eight-cell stage there still was 1.3-fold more laminin::mCherry at the gap edge compared with a similar region over the B1 cells ( Fig. 6a–c ; Supplementary Fig. 7e,f ; n =14, P <0.002, Student’s t test). Localization of INA-1,PAT-3::GFP was reduced at the vulval cell–BM gap boundary during E and F divisions (late P6.p four- and six-cell stages; Supplementary Fig. 7b,c ), but became increased in the vulD precursors when the BM stabilized over the course of the early and mid P6.p eight-cell stage ( Supplementary Fig. 7d,e ). At this time, we detected a ∼ 2.4-fold increase in INA-1,PAT-3::GFP at the D cell–BM interface ( Fig. 6a ) as compared with the divided F cells ( Fig. 6b,c ; n =14; P <1.0e-07, Student’s t test) or the B1 cells ( Fig. 6a,c ; Supplementary Fig. 7e,f ; n =14; P <1.0e-06, Student’s t test). Together, these results demonstrate that increased levels of laminin concentrate at the BM gap edge and correlate with enrichment of integrin through a post-transcriptional mechanism. 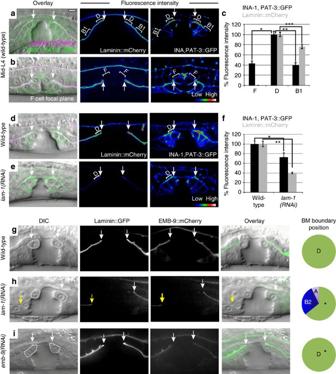Figure 6: Increased laminin at the edge of the BM opening promotes integrin localization. (a–f) DIC micrographs (left) and corresponding confocal sections depicting the fluorescence intensity as a spectral representation of integrin (INA-1, PAT-3::GFP, middle) and the BM (laminin::GFP, right) in wild-type (a,b,d) as compared withlam-1(RNAi)-treated animals (e). White arrows delineate the BM gap. (c,f) Quantification (shown as mean±s.e.m.) of 3.375 μm line scans (white brackets) of the fluorescence intensity of INA-1, PAT-3::GFP and laminin::mCherry at the vulval cell–BM interface at the mid-L4 stage (late P6.p eight-cell stage). (c)n=14 cases observed; *P<1.0e−06;**P<1e−07;***P<0.002, Student’sttest). (f)n=10 (wild-type) andn=18 (lam-1(RNAi)) cases observed; *P<0.01; **P<0.0001; Student’sttest). (g–i) DIC micrographs (left) and corresponding confocal sections of laminin::GFP (middle), EMB-9::mCherry (right) and overlay (far right). Pie charts depict BM gap position,n=20 (wild-type),n=28 (lam-1(RNAi)) andn=20 (emb-9(RNAi)) cases observed for each, seeSupplementary Fig. 8for BM gap measurements andSupplementary Table 2dfor scoring data. Yellow arrow depicts BM gap expansion beyond D cell (dashed line). *P<0.003;n=28 Fisher’s exact test as compared with wild-type (n=20). Scale bar, 5 μm. Figure 6: Increased laminin at the edge of the BM opening promotes integrin localization. ( a – f ) DIC micrographs (left) and corresponding confocal sections depicting the fluorescence intensity as a spectral representation of integrin (INA-1, PAT-3::GFP, middle) and the BM (laminin::GFP, right) in wild-type ( a , b , d ) as compared with lam-1 ( RNAi )-treated animals ( e ). White arrows delineate the BM gap. ( c , f ) Quantification (shown as mean±s.e.m.) of 3.375 μm line scans (white brackets) of the fluorescence intensity of INA-1, PAT-3::GFP and laminin::mCherry at the vulval cell–BM interface at the mid-L4 stage (late P6.p eight-cell stage). ( c ) n =14 cases observed; * P <1.0e−06; **P <1e−07; ***P <0.002, Student’s t test). ( f ) n =10 (wild-type) and n =18 ( lam-1(RNAi )) cases observed; * P <0.01; ** P <0.0001; Student’s t test). ( g – i ) DIC micrographs (left) and corresponding confocal sections of laminin::GFP (middle), EMB-9::mCherry (right) and overlay (far right). Pie charts depict BM gap position, n =20 (wild-type), n =28 ( lam-1(RNAi )) and n =20 ( emb-9(RNAi )) cases observed for each, see Supplementary Fig. 8 for BM gap measurements and Supplementary Table 2d for scoring data. Yellow arrow depicts BM gap expansion beyond D cell (dashed line). * P <0.003; n =28 Fisher’s exact test as compared with wild-type ( n =20). Scale bar, 5 μm. Full size image Given the correlation of increased laminin with integrin localization at the stabilized BM gap, we next tested whether the concentrated laminin might direct integrin here. Consistent with this notion, we detected a 27% reduction in INA-1,PAT-3::GFP at the D cell–BM interface following RNAi depletion of the sole β subunit of laminin, lam-1 , as compared with wild-type animals ( Fig. 6d–f ; n ⩾ 10 animals for each, P <0.01, Student’s t test). Strikingly, laminin depletion also caused BM gap overexpansion, as visualized by both laminin::GFP and EMB-9::mCherry (type IV collagen; Fig. 6h ), 36% of the time by the mid-L4 stage (10/28 cases of overexpansion past the D cell including two cases over the A cells, P <0.003; Fisher’s exact test; Fig. 6h ; Supplementary Fig. 8 and Supplementary Table 2d ). RNAi depletion of type IV collagen ( emb-9 ) failed to cause a BM gap overexpansion defect (20/20 cases, Fig. 6i ; Supplementary Figs 8 and 9a–c ), indicating that the overexpansion defect was specific to loss of laminin. Together, these results suggest that higher levels of laminin at a BM gap edge promotes increased surface integrin, which adheres to and stabilize the position of the gap edge. Integrin accumulates at the non-dividing F cell–BM gap edge The dependency of integrin on increased laminin localization suggested that this might be a flexible mechanism to stabilize BM gap boundaries on non-dividing cells. Thus, we next determined whether integrin levels increased at the F cell–BM boundary when F cell divisions were blocked ( cdh-3 >CKI-1::GFP; Fig. 5 ). Consistent with an inducible adhesion system, in cases where the BM stabilized over a non-dividing F cell we detected a significant 2.7-fold increase in levels of INA-1, PAT-3::GFP as compared with wild-type divided F cells ( Supplementary Fig. 9d–f ; n =14; P <1.0e−09, Student’s t test). These results suggest that increased integrin levels localize to the edge of the expanding gap on non-dividing vulval cells in response to laminin accumulation, thus providing an adaptive adhesion system to detect and stabilize BM gaps on non-dividing cells. Large gaps in BM occur in many developmental processes as well as metastatic cancer [2] , [6] , [8] , [16] , [46] . There has been significant progress on understanding the molecular and cell biological mechanisms that regulate BM breaching by invasive cells [16] ; however, little is known about how BM gaps might expand and stabilize their position. Understanding how BM openings are regulated is important, as large gaps facilitate morphogenetic movements and cell migration in development, and correlate with and might even stimulate metastatic cancer progression [11] , [47] , [48] . Here, we examine the evolution of rhabditid nematode uterine–vulval attachment and combine this with functional analyses within C. elegans to describe a new mechanism of targeted cell cycle regulation that expands and stabilizes BM gaps (summarized in Fig. 7 ). 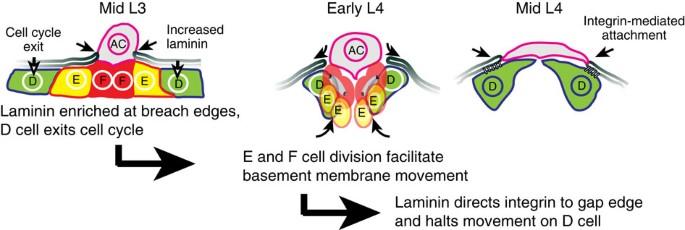Figure 7: Timed invasion, cell cycle regulation and laminin/integrin interactions initiate, expand and stabilize BM breaches. Schematic diagram depicting a model for initiation, opening and stabilization of the BM gap during uterine–vulval attachment. During the mid-L3 stage at the P6.p four-cell stage the D cells exit the cell cycle and increased laminin accumulates at the BM gap edge. In the early L4 stage the interior E and F cells divide, reduce contact with the BM, and the BM gap widens, driven by forces from the invaginating vulval cells that shift the BM freed from the dividing vulval cells. In the mid-L4 stage, laminin directs integrin to the gap edge, stabilizing the BM gap over the post-mitotic D cells. Figure 7: Timed invasion, cell cycle regulation and laminin/integrin interactions initiate, expand and stabilize BM breaches. Schematic diagram depicting a model for initiation, opening and stabilization of the BM gap during uterine–vulval attachment. During the mid-L3 stage at the P6.p four-cell stage the D cells exit the cell cycle and increased laminin accumulates at the BM gap edge. In the early L4 stage the interior E and F cells divide, reduce contact with the BM, and the BM gap widens, driven by forces from the invaginating vulval cells that shift the BM freed from the dividing vulval cells. In the mid-L4 stage, laminin directs integrin to the gap edge, stabilizing the BM gap over the post-mitotic D cells. Full size image Our comparative approach characterized several key events associated with nematode uterine–vulval attachment across 21 species of rhabditids, which last shared a common ancestor ∼ 280–430 million years ago [20] , [21] , [30] . First, we found that in all species examined, there is only a single AC, and in its absence, no other cell is capable of initiating a BM breach. This suggests that there is a strong selective pressure for the presence of only one AC, possibly to precisely control the timing or position of BM breaching. We speculate that this function may preclude later AC divisions that could help open the BM gap. Second, we have found in the sampled taxa that the timing of AC invasion occurs in a continuous distribution with a BM breach first observable in some species before P6.p division and in others not until the division of the daughters of P6.p cell (P6.p four-cell stage). Similar to many characters of vulval development in rhabditids [20] , [24] , [25] , [26] , [27] , [28] , we detected convergent or parallel changes in the timing of AC invasion, as AC invasion occurred at the late P6.p two-cell/early four-cell stage in two non-sister taxa Oscheius species ( O. dolichuroides and O. myriophila , phylogeny depicted in Supplementary Fig. 3 ) [22] . Notably, in all species examined, the initial breach in the BM occurred before vulval cell invagination. This suggests that there is selective pressure on the AC to breach the BM before invagination. One strong candidate for this evolutionary pressure is the necessity to make an initial BM breach before forces are generated by the invaginating and dividing VPCs that expand the gap. Consistent with this idea, we have observed that in AC invasion mutants in C. elegans with delayed timing of invasion (that is, post invagination), that the BM gap opening is narrow and does not move over the D cells ( Supplementary Fig. 10 ). Using laser ablation we also found that the AC is required to initiate the BM breach in all rhabditid species examined. This suggests that the AC may have evolved specifically to breach gonadal and ventral epidermal BMs and initiate uterine–vulval attachment. Interestingly, not all aspects of AC biology are conserved. For example, the induction of vulval cell fates, a key aspect of vulval patterning by the AC in C. elegans , is a derived feature within the Caenorhabditis nematodes, as many species show vulval induction earlier in gonad development via the lineage that gives rise to the AC and in some species vulval induction is even gonad independent [20] , [25] , [49] . Thus, our data strongly suggests that the AC’s role in initiating uterine–vulval attachment through BM invasion was selected for early in nematode evolution and may be a shared, derived character or synapomorphy of rhabditid nematodes. Our evolutionary and comparative studies also suggest that the process of active cell division helps expand BM openings and that non-dividing cells stabilize gap edges. Following AC invasion in C. elegans , the vulval cells undergo a period of expansion, invagination and division. These morphogenetic processes are thought to provide the mechanical force to move the overlying BM [13] . We show here that actively dividing E and F cells reduce contact with the BM, and that cell division followed by loss or reduction of attachment provides a mechanism to allow movement of the BM edge onto the neighbouring non-dividing D cell. Supporting this model, we find that inhibition of E and F cell divisions halts BM movement and limits gap expansion. Previously, a large-scale comparative analysis of nematode vulval development identified the D cell as the only vulval cell that never divides following the P6.p four-cell stage across all surveyed rhabditid nematodes [20] . Our data provide compelling evidence that cell cycle exit of the D cell may have been maintained over 300 million years of nematode evolution to stabilize the position of the BM gap. Further supporting this notion, we observed that the BM gap stabilizes over the E cells in the Mesorhabditid Bursilla sp ., which has undergone a natural loss of the final E cell division [20] . Controlled cell cycle regulation might be a common strategy for positioning BM gap openings, as actively dividing cells are known to lose BM adhesions, including hemidesmosomes [50] . This may be especially important with cells undergoing epithelial to mesenchymal transition, where large but specific gaps in BM helps define fundamental germ layer, tissue and organ boundaries [5] , [6] , [51] . Loss of control over division might also inappropriately promote expansion of BM breaches in growing tumours, which might enhance malignancy [9] , [52] . How BM gaps may be detected for stabilization is unknown. Our results indicate that the BM gap edge itself provides a signal for stabilization. The invading AC displaces BM, and this results in enriched laminin at the edges of the initial BM breach [19] . We show that this increased laminin persists during gap expansion and corresponds precisely with increased localization of the integrin heterodimer INA-1/PAT-3, which stabilizes the BM gap position. Further, we find that depletion of the β subunit of laminin ( lam-1 ) by RNAi results in a decrease in integrin localization at the BM gap edge and a gap overexpansion defect. Notably, ina-1 is thought to be most similar to laminin-binding integrins [44] , [45] , [53] , suggesting a direct interaction between laminin and INA-1/PAT-3. Together, our results support a hypothesis where increased laminin at the BM gap edge recruits INA-1/PAT-3 integrin, which acts to stabilize the position of the BM gap over the non-dividing vulD precursors. Intriguingly, invasive cancer cells and epithelial cells have been shown in vitro to generate compression forces that similarly displace BM, which accumulates at edges of holes generated in matrix [54] , [55] . Furthermore, podosomes, which are invasive subcellular structures that contact and remodel BM, generate outward forces, that may displace BM [56] . Thus, edges of BM gaps might often accumulate laminin and upregulate integrin to stabilize breaches in BM. Our combined cell, developmental and evolutionary results provide a model for how a de novo gap in the BM is opened, expanded and then stabilized. Following BM breaching from an evolutionarily conserved invasive cell, the AC, we show that active cell division during invagination allows the BM to move, thus widening the gap. We also demonstrate that cell cycle exit leads to laminin-directed adhesion that stabilizes BM gap opening ( Fig. 7 ). The highly collaborative interactions that direct the precise opening in the BM during uterine–vulval connection likely evolved to facilitate direct interactions between specific uterine and vulval cells that form the mature attachment. Similar interactions between invasive cells and tissues might be a hallmark of BM gap formation during many other developmental processes and tumour progression where active cell division, growth and tissue expansion impose dynamic forces that can shift and stabilize BM openings. Strains and culture conditions Rearing and handling conditions of all 21 species of rhabditid nematodes, including C. elegans , was done as previously described for C. elegans [57] . Wild-type C. elegans animals were strain N2. For a list of strain designations for the other 20 nematode species see Supplementary Table 1 . In the text and figures, we refer to linked DNA sequences that code for a single fusion protein using a double colon (::) annotation. For designating linkage to a promoter we use a greater than symbol (>). The following alleles and transgenes were used in this study: weEx70[cdt-2::GFP] , rhIs2[pat-3::GFP] [58] , qyIs232[cdt-1::GFP] , qyIs229[cdh-3>H2B::GFP] , qyIs110[egl-17>HA-β-tail] [13] , qyIs330[laminin::mCherry] , qyIs351 [unc-62>GFP::CAAX] ; LGI: ayIs4 [egl-17>gfp] ; LGIV: qyIs10[laminin::GFP] , qyIs42[genomic ina-1,pat-3::GFP] [42] ; LGV: qyIs127[laminin::mCherry] , qyIs266 [cdh-3>cki-1::GFP] ; LGX: qyIs46[emb-9::mCherry] , qyIs7[laminin::GFP] . Microscopy image acquisition and processing Except where noted, confocal images were acquired using a CCD digital camera (OrcaR2 Hamamatsu Photonics) and a spinning disk confocal microscope (CSU-10; Yokogawa) mounted on a compound microscope (Axioimager; Carl Zeiss) with a Plan-APOCHROMAT × 100/1.4 oil differential interference contrast objective and controlled by either iVision software (Biovision Technologies) or μManager [59] . All other images were acquired using a CCD digital camera (Axiocam mrm; Carl Zeiss) mounted on a microscope (Axioimager; Carl Zeiss) with a Plan-APOCHROMAT × 100/1.4 oil differential interference contrast objected controlled by either Axiovision 4.6 (Carl Zeiss) or Zen 2012 (Carl Zeiss). Acquired images were processed using ImageJ 1.46r and Photoshop (CS5.1; Adobe). For microscopy, worms were anaesthetized on 5% agar pads containing 0.01 M NaN 3 . To avoid bias, for each individual experiment, images were acquired in a random order. Data analyses Individual data points for each experiment were collected over multiple days and for those experiments involving RNAi knockdown, included data from multiple RNAi treatments. For each experimental condition, no image that corresponded to the correct state was excluded from our analyses. For quantitative analyses, images were first normalized by default background subtraction in Image J. Quantitative analyses of integrin (INA-1, PAT-3::GFP) and laminin (laminin::GFP or laminin::mCherry) localization was done in Image J using a 5-pixel line scan and the plot profile function to quantify fluorescence intensity as a function of distance. The average of the fluorescence intensity of these transgenes across multiple animals over a 3.375 μm distance (representing the region of contact between the vulval cell and the overlying BM) from the plot profile (data shown in Supplementary Fig. 7 ) was used to generate the average fluorescence intensity. For analysis of wild-type fluorescence intensity measurements were repeated twice using two different laminin::mCherry transgenes (qyIs127 and qyIs330) paired with the same integrin (INA-1,PAT-3::GFP) transgene (qyIs42). BM gap edge to vulval midline measurements were done in Image J. Figures and graphs were constructed using Illustrator (CS5.1; Adobe). Dextran injections To visualize the BM during vulval development rhodamine-labelled dextran was injected into the body cavity of L3 and L4 stage animals of C. elegans strain NK248 ( qyIs10[laminin::GFP] ), Oscheius carolinensis YEW1, Pristioncus pacificus PS132 and Bursilla sp. PS1179. Animals were recovered following injection and imaged as described above (see Microscopy section). The C. elegans strain containing a laminin::GFP transgene (qyIs10) was injected with rhodamine dextran to confirm that dextran colocalized to the BM ( Supplementary Fig. 2a ). AC ablations Laser-directed cell ablations of the AC in C. elegans and the other 20 species of rhabditid nematodes were carried out on 5% agar pads as previously described [17] , [60] . Briefly, a laser combination system (using a nitrogen and dye laser with a 5 mM coumarin 120 dye in ethanol) generates nanosecond length pulses of 440 nm light, which is focused on the desired cell using a Zeiss Axioskop microscope (Carl Zeiss) with a × 100 DIC objective [60] . Between 10 and 25 laser bursts were used to kill each AC. Ablated animals were recovered from the agar pad, allowed to develop at 20 °C until the mid-L4 stage and then examined for AC invasion defects and an intact BM. A minimum of 10 ACs were ablated for each species. Construction of GFP and mCherry protein fusions A 5.9-kb fragment containing the entire cdt-1 genomic region before its stop codon was amplified from N2 genomic DNA and then linked to GFP amplified from pPD95.75 by PCR fusion. H2B::GFP was amplified from pLZ6 and then linked to a ∼ 5-kb fragment of the cdh-3 promoter by PCR fusion. Cki-1::GFP was amplified from a recombineered fosmid WRM0626bF02 (wTRG5.1_2491680425634929_G10) and linked to a ∼ 5-kb fragment of the cdh-3 promoter by PCR fusion. GFP::CAAX was amplified from pSA129, and then linked by PCR fusion to the unc-62 promoter. Constructs were coinjected with 50 ng μl −1 unc-119 rescue DNA, ∼ 50 ng μl −1 pBsSK and 25 ng μl −1 EcoRI cut salmon sperm DNA into unc-119(ed4) hermaphrodites. Multiple stably expressing extrachromosomal lines were established and selected lines were integrated by gamma irradiation. See Supplementary Tables 3 and 4 for transgenic strains generated and primer sequences used. RNA interference Double-stranded RNA (dsRNA) used in this study was delivered by feeding to strains containing the following transgenes: qyIs229[cdh-3>H2B::GFP], qyIs127[laminin::mCherry]; qyIs46[emb-9::mCherry], qyIs10[laminin::GFP]; qyIs42[ina-1,pat-3::GFP], qyIs330[laminin::mCherry]; qyIs110[egl-17>HA-β-tail], ayIs4[egl-17>GFP] and qyIs127[laminin::Cherry] . RNAi feeding of starved L1 stage animals was performed following synchronization using hypochlorite treatment of gravid adults and phenotypes were scored at the L4 stage. The RNAi vector targeting cul-1 is from the Vidal RNAi library [61] and the RNAi vectors targeting lam-1 (laminin β subunit) and emb-9 (type IV collagen) are from the Ahringer RNAi library [62] . The empty vector L4440 was used as a negative control. The RNAi vectors for cul-1 , lam-1 and emb-9 were verified by sequencing. Statistical analysis For fluorescence quantification analyses sample size was validated a posteriori for variance and statistical significance. The variance was similar within each experimental data set, as assessed for normality using a Shapiro–Wilk’s normality test for each data series. Statistical analyses were performed using either a two-tailed unpaired Student’s t test or the Freemon–Halton extension of the Fisher’s exact probability test for a two-rows by three-columns contingency table. Figure legends specify when each test was used and whether the error bars represent s.d. or s.e.m. For all statistical tests P <0.05 was considered significant. How to cite this article: Matus, D. Q. et al . Cell division and targeted cell cycle arrest opens and stabilizes basement membrane gaps. Nat. Commun. 5:4184 doi: 10.1038/ncomms5184 (2014).